In-gap quasiparticle excitations induced by non-magnetic Cu impurities in Na(Fe0.96Co0.03Cu0.01)As revealed by scanning tunnelling spectroscopy The origin of superconductivity in the iron pnictides remains unclear. One suggestion is that superconductivity in these materials has a magnetic origin, which would imply a sign-reversal s ± pairing symmetry. Another suggests it is the result of orbital fluctuations, which would imply a sign-equal s ++ pairing symmetry. There is no consensus yet which of these two distinct and contrasting pairing symmetries is the right one in iron pnictide superconductors. Here we explore the nature of the pairing symmetry in the superconducting state of Na(Fe 0.97− x Co 0.03 Cu x )As by probing the effect of scattering of Cooper pairs by non-magnetic Cu impurities. Using scanning tunnelling spectroscopy, we identify the in-gap quasiparticle states induced by the Cu impurities, showing signatures of Cooper pair breaking by these non-magnetic impurities–a process that is only consistent with s ± pairing. This experiment provides strong evidence for the s ± pairing. Since the discovery of high-temperature superconductivity in the iron pnictides [1] and chalcogenides [2] in early 2008, the pairing mechanism remains unsolved yet. The sensitivity of electronic band structure to the tiny change of structural parameters and the multi-band property make it very difficult to settle down this problem [3] . The quantum critical point located in the optimum doping level [4] in iron-based superconductors confirms the close relationship between superconductivity and antiferromagnetism. It was proposed that the binding force between the two electrons of the Cooper pair might be established through the magnetic origin, either by exchanging the anti-ferromagnetic spin fluctuations [5] or through local magnetic interactions, and consequently the electron and hole pockets should have s -wave gap with opposite signs (the s ± pairing scenario) [6] , [7] . As far as we know, there are no experiments that give direct evidence to support the s ± model. This gap structure gets support from the scanning tunnelling spectroscopy (STS) and the quasiparticle interference measurements in Fe(Se,Te) (ref. 8 ), in which a unique Q 2 interference spot was observed reflecting the quasiparticles (QPs) induced by the non-magnetic impurities within the s ± pairing model. Another indirect evidence was given by the observation of the resonance peak of the imaginary part of the spin susceptibility at ( π , π ) in the inelastic neutron scattering experiment [9] . In the case of s ± pairing, although there is a sign reversal of the gap, because the individual Fermi surface is fully gapped, one may not be able to detect it through the phase-sensitive experiment as conducted in the cuprate superconductors (ref. 10 and references therein). Alternatively, one can detect this unique pairing model through the impurity effect. In the superconducting state, the impurities may induce the QP scattering, break Cooper pairs and generate a unique pattern of the local density of states (LDOS) of QPs. This pattern is sensitively dependent on the pairing gap structure and the characteristics of the impurities [11] , [12] . According to the Anderson’s theorem [13] and the subsequent calculations [11] , [12] , [14] , [15] , [16] , the Cooper pairs with a uniform singlet superconducting gap structure (for example, the s -wave gap) can survive in the presence of non-magnetic impurities, whereas the magnetic impurities are very detrimental to superconductivity yielding a unique pattern of the QP-LDOS. This impurity state, after the pioneer work of Yu–Shiba–Rusinov [14] , [15] , [16] , has been well proved in the conventional superconductor Nb by the STS measurements using Mn adatoms as the magnetic scattering centres [17] . In the cuprate superconductors, when doping Zn atoms (the usually believed non-magnetic impurities) to the Cu sites, the superconductivity is suppressed greatly and a strong peak of the LDOS is observed near bias zero energy at the Zn impurity, which suggests an unconventional pairing symmetry and an anomalous normal state [18] . Theoretically it was argued that the s ± type pairing should be also fragile to the non-magnetic impurities when the scattering potential ( V imp ) is moderate ( V imp ≥1 eV) [19] , [20] , [21] , [22] , [23] , [24] , namely the in-gap QP excitations should be observable. However, some experiments show a slow suppression rate of superconducting transition temperature to impurity scattering, which seems to violate the Anderson’s theorem and leads to the conjecture of the s ++ pairing [19] . Furthermore, a picture of orbital-fluctuation-mediated superconductivity was proposed based on the analysis of five orbital Hubbard–Holstein model, which predicts an s ++ pairing [25] . In fact, the spatial and energy-dependent LDOS induced by the impurity scattering are very essential for having a formal check on the pairing model of s ± or s ++ . In previous STM studies, impurities have been successfully located in iron pnictide superconductors and many interesting features have been reported (refs 26 , 27 , 28 , 29 , 30 , 31 , 32 , and T. Hanaguri, et al. , private communications). However, it remains to be a great challenge to figure out which impurities are magnetic or non-magnetic. It is highly desired to locate a well-defined quantum impurity, prove by experiment whether they are magnetic or non-magnetic and investigate the related LDOS at and nearby the impurity. It becomes vital to pin down the s ± pairing model by observing the in-gap QP states induced by the non-magnetic impurities. In our previous study, we identified the Co impurities and found that the spatial evolution of the STS crossing a Co impurity in Na(Fe 1− x Co x )As is weak and not obvious [31] , which is explained in the picture that the Co impurity may give a weak and extended scattering potential, induces mainly the intra-pocket scattering and thus cannot significantly break the Cooper pairs assuming that the pairing is established by the inter-pocket scattering. Here we demonstrate the STS data obtained on Na(Fe 0.96 Co 0.03 T 0.01 )As single crystals with T=Mn ( T c ≈12.8 K) and Cu ( T c ≈16.0 K). Our DC magnetization measurements indicate that the Mn dopants will contribute magnetic, whereas the Cu dopants give rise to non- or very weak magnetic impurities. (Concerning the magnetic moments of Cu impurities, it cannot be precisely regarded as non- or weak magnetic; however, the DC magnetization signal here tells that the Cu doping gives rises to a value even weaker than the background. In this case, we naturally regard them as the non-magnetic centres.) However, strong in-gap QP DOS are clearly observed for either Cu or Mn impurities. Our results, especially the observation of the in-gap QP states by the non-magnetic Cu impurities, give decisive evidence for the sign-reversal gap structure, that is, the s ± pairing in the present samples. 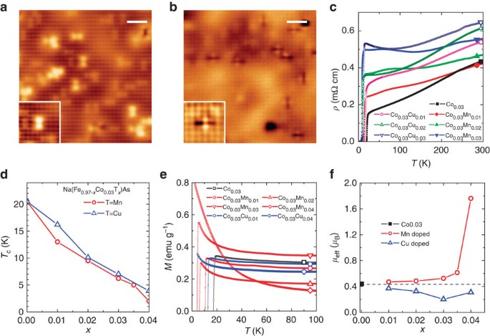Figure 1: Topographic STM images and characterizations of the related single crystals (a,b) STM images of the Cu-doped and the Mn-doped samples with the a bias voltage ofVbias=15, 8 mV and tunneling current ofIt=100, 150 pA, respectively. The inset shows the rescanned data in a small area with much higher pixel, from which one can clearly see the Cu and Mn impurities. (a,b) Scale bars, 2 nm. (c) Temperature dependence of resistivity for the pristine sample and the doped ones. The superconductivity is suppressed clearly when the residual resistivity is enhanced. (d) The doping dependence of the critical transition temperatureTcfor both the Cu- and Mn-doped samples. (e) The magnetization measured atμ0H=1T on the pristine sample (black open squares), the Cu-doped samples (blue symbols) and the Mn-doped samples (red symbols). One can see that the low temperature up-turn gets enhanced clearly by the Mn doping, but not enhanced by the Cu doping. (f) The average magnetic moment per Fe site calculated by the Curie–Weiss law for the Cu- and Mn-doped samples. Clearly, doping Mn induces strong averaged magnetic moments, whereas doping Cu seems to weaken the averaged local moments. Identification of the dopant atoms Figure 1a,b present the topographic images of the cleaved surfaces with the orientation (001) of Cu- and Mn-doped single crystals Na(Fe 0.96 Co 0.03 T 0.01 ) As (T=Cu and Mn). In the Na(Fe 1− x Co x )As system, the optimal doping is achieved around x =0.03 with superconducting transition temperature T c =20.5 K. Further doping of Cu and Mn to the Fe site is achieved starting from the status of this pristine sample. In the Cu-doped samples, in addition to some 3 × 2 blocks with light bright colour, as we discovered in the pristine Co-doped samples [31] , one can clearly see some extra spots with a dumbbell shape and much stronger brightness. The former are corresponding to the Co-doped sites, as we described clearly in previous paper [31] , the latter are the impurity sites induced by the Cu atoms. The two different orientations of these dumbbells for the Cu impurities have the same origin as the Co impurities, mainly been induced by the selective substitution to the Fe site which is surrounded by six Na atoms on the top layer. We illustrated this in Supplementary Note 1 . A scan with a much higher pixel was taken and the data are shown for the region near a Cu impurity in the inset of Fig. 1a . A close scrutiny finds that the brightness of the dumbbell decays actually in a scale of about 15–20 angstrom, being much larger than the Co impurity, which will be further corroborated by the spatial evolution of the LDOS. In the Mn-doped samples, since the topographic image was taken with a lower voltage (8 meV), the Co sites are barely visible. However, we clearly see some spots with a dark-bright crossing pattern. As amplified in the inset of Fig. 1b , the dark bar seems to be slightly longer than the bright wing. Clearly the Mn impurity gives a very different pattern of image compared with the Cu impurity. Qualitatively one may categorize the Co and Cu impurities as the same type, namely non- or weak magnetic, as they have quite similar shapes of topographic image. This will be corroborated by the DC magnetization measurements illustrated below. The reason for different patterns of images between Cu (also Co) and Mn dopants remains unresolved yet and is highly desired for further theoretical input. Figure 1: Topographic STM images and characterizations of the related single crystals ( a , b ) STM images of the Cu-doped and the Mn-doped samples with the a bias voltage of V bias =15, 8 mV and tunneling current of I t =100, 150 pA, respectively. The inset shows the rescanned data in a small area with much higher pixel, from which one can clearly see the Cu and Mn impurities. ( a , b ) Scale bars, 2 nm. ( c ) Temperature dependence of resistivity for the pristine sample and the doped ones. The superconductivity is suppressed clearly when the residual resistivity is enhanced. ( d ) The doping dependence of the critical transition temperature T c for both the Cu- and Mn-doped samples. ( e ) The magnetization measured at μ 0 H =1T on the pristine sample (black open squares), the Cu-doped samples (blue symbols) and the Mn-doped samples (red symbols). One can see that the low temperature up-turn gets enhanced clearly by the Mn doping, but not enhanced by the Cu doping. ( f ) The average magnetic moment per Fe site calculated by the Curie–Weiss law for the Cu- and Mn-doped samples. Clearly, doping Mn induces strong averaged magnetic moments, whereas doping Cu seems to weaken the averaged local moments. Full size image STS results crossing a non-magnetic Cu impurity Although the topographic images of the Cu and Mn impurities are very different, they however suppress the superconductivity in a similar way. In Fig. 1c , we present the temperature dependence of resistivity of the pristine sample Na(Fe 0.97 Co 0.03 )As with T c =20.5 K, and the Mn- and Cu-doped samples with doped concentration of 1%, 2% and 3%. One can see that the superconducting transition temperature drops down with the increase of doping as well as the residual resistivity. Interestingly, the suppression rate of Δ T c /Δ x (as shown in Fig. 1d ) is quite close to each other for the two doping ways. For evaluating the magnetic moments induced by these dopants, we present in Fig. 1e the temperature dependence of DC magnetization measured at μ 0 H =1 T for several typical samples. The magnetization hysteresis loops measured on these samples clearly show a reversible, roughly linear and paramagnetic background above 2 K. Therefore, we naturally assume that the magnetization can be written in the Curie–Weiss law, χ = M / H = χ 0 + C 0 /( T + T θ ), where , χ 0 and T θ are the fitting parameters, μ eff is the local magnetic moment per Fe site. The first term χ 0 comes from the Pauli paramagnetism of the conduction elections, which is related to the DOS at the Fermi energy. The second term C 0 /( T + T θ ) is contributed by the local magnetic moments given by the Fe sites (including Co, Cu and Mn). In this way, by adjusting the χ 0 value, we should be able to get a linear function of 1/(χ−χ 0 ) versus T in the low temperature region. Then we fit the data with a linear function, the slope gives 1/C 0 , and the intercept provides the value of T θ /C 0 . Once C 0 is obtained, we can get the average magnetic moment of a single Fe site (including the contribution of Fe and the dopants Cu, Mn and Co). For the pristine sample (3% Co-doped), the magnetization shows a very weak up-turn in the low temperature region indicating a weak magnetic moments per Fe. With the doping of Cu, no enhancement of the up-turn at low temperatures is observed. This is in sharp contrast with the Mn-doped samples, one can see that the up-turn at low temperatures is clearly getting enhanced with the increase of the doped Mn concentration. In order to get a quantitative assessment on the magnetic moments, we fit the data below 40 K for all samples based on the Curie–Weiss law mentioned above and present the results in Fig. 1f . It is clear that Cu-doping seems to lower down the averaged magnetic moments, whereas Mn-doping gives rise to a continuing increase of the local magnetic moments. As the measured average magnetic moment after doping Cu is even slightly lower than the pristine sample, this suggests that the Cu impurity may diminish the local magnetic moments. One possible picture to interpret this is that the Cu dopant may have a full shell of electrons with the ionic state of Cu 1+ as predicted by the first-principles calculations [33] and the density functional calculation [34] . All these facts justify that we can categorize the Cu dopants as the non- or very weak magnetic impurities. We should mention that doping Cu in the present FeAs-based samples and doping Zn in the cuprates may have different effect. In the latter case, it was supposed that the Zn doping in the cuprate superconductors would remove a spin causing a background magnetic correlation near the Zn impurity. This may induce a strong magnetic moment near the Zn impurity and thus produce the huge impurity peak in the tunnelling spectrum [18] . This does not seem to be the case in the present Cu-doped Na(Fe 0.97− x Co 0.03 Cu x )As samples as the susceptibility derived in our bulk magnetic measurements do not indicate an enhanced magnetic moment. However, more local measurements are still worthy of doing for checking the weakened or diminishing of the local magnetic moments by doping Cu. For the Mn dopants, however, they certainly behave as the magnetic impurities here. In Fig. 2a , we show the topographic image around the single Cu impurity. After identifying the Cu impurity and confirming that they are non-magnetic impurities, we measure the STS by crossing one single Cu impurity with steps of half Na–Na lattice constant ( a 0 /2) with a 0 ≈3.85±0.05 Å, and show them in Fig. 2c . A gradual evolution of the tunnelling spectra can be easily seen here. At a distance of about 2 nm away, the STS shows a typical superconducting one with two clear coherence peaks at about ±5 meV. This energy gap is well consistent with the values derived from the angle-resolved photo-emission measurements [35] . There is a lifted height on the STS near zero bias energy even when it is far away from the impurities, this may be caused by two reasons: (1) doping Cu can induce the in-gap QP excitations, even it is far away from the impurity site; (2) the measuring temperature is 1.7 K, which may induce some thermal broadening effect and lift the conductivity at zero bias energy. When approaching the impurity site of Cu (the centre of the dumbbell shape of the image), the coherence peak on the negative-biased voltage is strongly suppressed and the one on the positive side shifts to a smaller voltage. The typical STS, measured at the Cu site and 2 nm away, respectively, at different temperatures, that is, in the superconducting state at 1.7 K (solid lines) and in the normal state at 17 K (dashed lines), are presented in Fig. 2b . In order to know how the Cu impurity gives the influence on the STS, we subtract the STS curves measured at different positions with that measured 2 nm away and present the results in Fig. 2d , one can clearly see that the difference of the STS exhibits a huge asymmetric peak within the superconducting gap. This is very different from the case when crossing the Co site, there we did not see obvious spatial change of the STS [31] . We will discuss these unique in-gap states later. Furthermore, to check how strong the Cu impurity would affect the electronic properties spatially, we present the spatial mapping of the LDOS measured at different energies in Fig. 3b–f . One can see a systematic evolution of the LDOS around the Cu impurity with a spatial scale of about 1.5–2.0 nm. This scale is the same as the size of the dumbbell shape shown by the topographic image ( Fig. 2a ). Actually, the in-gap states exist in a spatial scale of about 4.5 a 0 =17.33±3 Å as can be seen in Fig. 2d . Assuming that the Cu impurity gives rise to a point disorder, the in-gap states may decay in a scale of the coherence length ξ . Therefore, one can roughly estimate the coherence length as ξ ≈17.33±3 Å, which is smaller than that determined in BaFe 1.8 Co 0.2 As 2 single crystals (~27.6 Å) [26] , [27] calculated from the structure of the vortex. This difference may be ascribed to the distinct superconducting gap Δ sc and the Fermi velocity v F in the two different systems, as ξ ∝ v F /Δ sc . An alternative explanation for the smaller coherence length derived here is that the measurements are done on the Na surface, the in-gap states measured on this surface would show up in a reduced spatial region compared with that if they would be measured directly on the Fe layer. 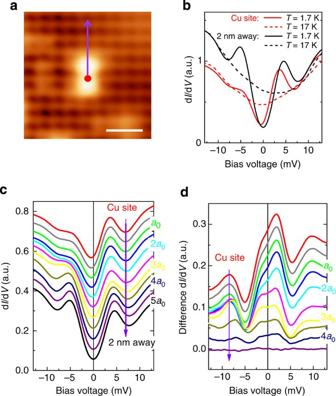Figure 2: Tunneling spectra at and near the Cu impurity. (a) The topographic image near a Cu impurity, the bright pattern with a dumbbell shape is corresponding to a Cu impurity. One can also see several Co impurities with lighter brightness. (a) Scale bar, 1 nm. (b) The STS measured at the Cu impurity (red line) and that measured 2 nm away (dark line). The dashed lines are the spectra measured at 17 K, and they can be used as the normal state background. (c) The STS measured at the Cu impurity (red line) and those measured with steps of every half Na–Na lattice constant on the surface. (d) The subtracted results of the STS with that measured at 2 nm away from the Cu site, the colours of the lines are the same in (c). The STS in (c,d) are off-set for clarity. One can easily see the emerging in-gap states when approaching the Cu impurity. Figure 2: Tunneling spectra at and near the Cu impurity. ( a ) The topographic image near a Cu impurity, the bright pattern with a dumbbell shape is corresponding to a Cu impurity. One can also see several Co impurities with lighter brightness. ( a ) Scale bar, 1 nm. ( b ) The STS measured at the Cu impurity (red line) and that measured 2 nm away (dark line). The dashed lines are the spectra measured at 17 K, and they can be used as the normal state background. ( c ) The STS measured at the Cu impurity (red line) and those measured with steps of every half Na–Na lattice constant on the surface. ( d ) The subtracted results of the STS with that measured at 2 nm away from the Cu site, the colours of the lines are the same in ( c ). The STS in ( c , d ) are off-set for clarity. One can easily see the emerging in-gap states when approaching the Cu impurity. 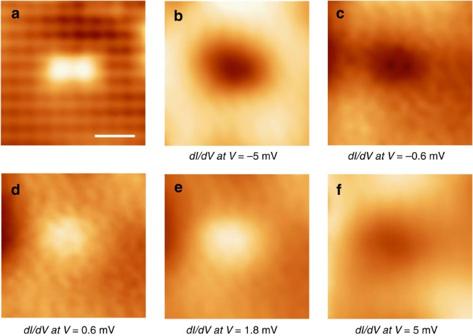Figure 3: Mapping of the LDOS measured near a Cu impurity. (a) The topographic image of a Cu impurity, the field of view dimensions are 3.5 × 3.5 nm. (a) Scale bar, 1 nm. (b–f) The mapping of the LDOS measured at bias voltages of −5, −0.6, 0.6, 1.8 and 5 mV, respectively. One can see that the spatial influence of a Cu impurity is about 20 Å. Full size image Figure 3: Mapping of the LDOS measured near a Cu impurity. ( a ) The topographic image of a Cu impurity, the field of view dimensions are 3.5 × 3.5 nm. ( a ) Scale bar, 1 nm. ( b – f ) The mapping of the LDOS measured at bias voltages of −5, −0.6, 0.6, 1.8 and 5 mV, respectively. One can see that the spatial influence of a Cu impurity is about 20 Å. Full size image Impurity states near a magnetic Mn dopant atoms For a comparison, we also measured the STS around a Mn impurity and presented the results in Fig. 4 . Now one can see that, even the measurement is done about 1.2 nm away from the Mn site, a very asymmetric STS can still be observed. This asymmetry may reflect the effect given by the impurity scattering which produces the QP-DOS near the gap edge. Therefore, the sharp peaks at the gap edges may be due to the merging of the superconducting coherence peak together with the impurity induced states. However, this type of asymmetric curve can be even seen at a distance far away from the Mn site, which may challenge the simple understanding mentioned above. When approaching to the Mn site, one can see that the sharp peaks near the superconducting gap become broadened and move gradually to higher energies. At the meantime, an in-gap peak appears around zero bias energy and is getting enhanced very near the Mn site. This in-gap peak is certainly derived from the QP excitations by the scattering effect of the Mn impurity, and it is no doubt that the Mn impurities are playing as the strong pair breakers. The interesting point is that the STS exhibits different evolutions along the dark bar and the bright wing on the image. The modification to the STS by the scattering effect shows up at 2 a 0 from the Mn site when measured along the dark bar, whereas it starts at about a 0 when along the bright wing. Moreover, the in-gap state peak seems to locate at or very near zero bias voltage when it is measured on the atom with enhanced brightness in the image. The detailed reason is still unknown and waits for further understanding. Clearly, either the non-magnetic Cu or the magnetic Mn impurities can induce in-gap QP excitations. 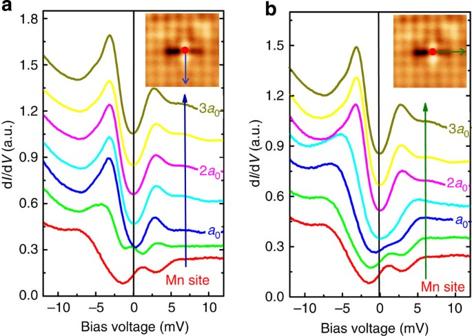Figure 4: The STS measured around a Mn impurity. (a,b) The STS measured at the Mn site (red line) and those measured with steps of every half Na–Na lattice constant on the surface, along the line of (a) bright-wing and (b) dark-bar on the images as shown in the insets. The shape of STS exhibits a strong evolution spatially, indicating a clear presence of the in-gap states. At the Mn site and the position one step away, one can see a peak of in-gap states directly from the STS, as shown by the red and green curves. Figure 4: The STS measured around a Mn impurity. ( a , b ) The STS measured at the Mn site (red line) and those measured with steps of every half Na–Na lattice constant on the surface, along the line of ( a ) bright-wing and ( b ) dark-bar on the images as shown in the insets. The shape of STS exhibits a strong evolution spatially, indicating a clear presence of the in-gap states. At the Mn site and the position one step away, one can see a peak of in-gap states directly from the STS, as shown by the red and green curves. Full size image Theoretical calculations To investigate the in-gap states from the non-magnetic impurity observed in our experiments, we do further theoretical calculations and compare with the experimental data. Details of the theoretical calculations are described in Supplementary Note 2 . The energy dispersion from the ab initio calculation is shown in Fig. 5a along high symmetry cuts, and compares well to that in the literature [34] , [35] . 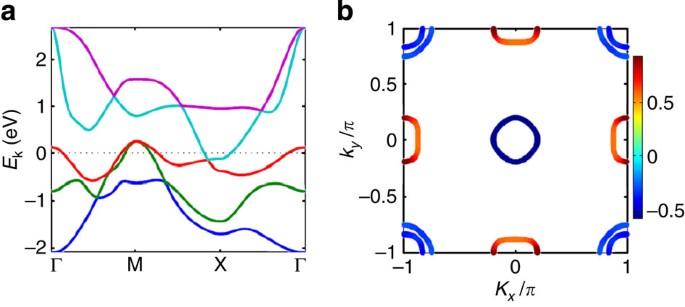Figure 5: Band structure and Fermi surface from theab initiocalculations. (a) Band structure along high symmetry cuts. (b) Fermi surfaces. The colour scale shows the sign and magnitude of the pairing function projected on the Fermi surfaces. Figure 5b shows the Fermi surface relevant to the material. In Fig. 6 we present the comparison between the experiment and the theoretical calculations for the Cu impurities. In order to have an effective comparison, we present here the data normalized by the normal state background, as shown in Fig. 6a . The normalized curves were obtained by dividing the data measured at 1.7 K with that at 17 K shown in Fig. 2b , respectively. On can see that the STS exhibits an elevated bottom at zero bias voltage, this is quite natural for the impurity-induced pair breaking and thermal broadening at a finite temperature. Interestingly, at the Cu site, the coherence peak at the positive bias seems moving inward indicating the suppression to the order parameter. In Fig. 6b , we show the difference of the STS measured at the Cu site and 2 nm away. The difference of these two STS shows a prominent peak near zero bias, with the sharp peak at a slight positive bias voltage (around 2 meV). It is interesting to mention that in the previous experiments on conventional Nb superconductor [17] , the magnetic impurity Mn gives a very similar effect. The only difference is that the sharp peak appears at a slightly negative voltage side there. Here we observe such peak with a non-magnetic impurity, which manifests itself that we should have a sign reversal on the superconducting gap. In order to corroborate this point, we did theoretical calculations and present the calculated results in Fig. 6c,d . Here we use a five-orbital band structure derived from ab initio calculations. Assuming local Coulomb and Hund’s rule interactions, we performed functional renormalization group calculations to get the best pairing gap function (which turns out to have s ± symmetry as expected), enabling us to write down an effective Hamiltonian describing the superconducting state. The effect of local impurity is then handled by the standard T-matrix formalism. More technical details and parameters in the calculation are described in Supplementary Note 2 . Figure 5: Band structure and Fermi surface from the ab initio calculations. ( a ) Band structure along high symmetry cuts. ( b ) Fermi surfaces. The colour scale shows the sign and magnitude of the pairing function projected on the Fermi surfaces. 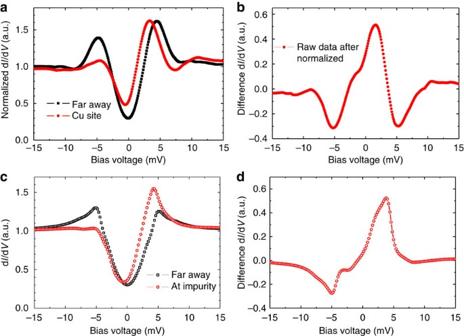Figure 6: Comparison between experiment and theory. (a) The tunneling spectrum measured at the Cu site (red-filled symbols) and that about 2 nm away (dark-filled symbols) normalized by the normal state background. (b) The difference between the two curves shown ina. (c) The STS obtained from the theoretical calculations at the scalar impurity (red open circles) and off the impurity site (dark open squares). (d) The difference between the two curves shown inc. One can see that the calculation can really reproduce the main structure of the measured data. A calculation with thes++model was tried and could not produce the in-gap states. Full size image Figure 6: Comparison between experiment and theory. ( a ) The tunneling spectrum measured at the Cu site (red-filled symbols) and that about 2 nm away (dark-filled symbols) normalized by the normal state background. ( b ) The difference between the two curves shown in a . ( c ) The STS obtained from the theoretical calculations at the scalar impurity (red open circles) and off the impurity site (dark open squares). ( d ) The difference between the two curves shown in c . One can see that the calculation can really reproduce the main structure of the measured data. A calculation with the s ++ model was tried and could not produce the in-gap states. Full size image There are two possible scenarios to interpret the impurity induced in-gap DOS observed in our experiment. The first is a pairing state with in-phase gap on all Fermi pockets ( s ++ pairing) but subject to magnetic impurities, as described for Mn in the conventional Nb superconductor [17] . This scenario can be ruled out here as no prominent magnetic signature is detected on the Cu impurities. The second is a pairing state with s ± pairing on electron/hole pockets subject to non-magnetic impurities. This is because a local impurity can scatter electrons both within and between the pockets. The inter-pocket scattering sees the sign reversal of the gap function (on electron and hole pockets), hence can induce in-gap states. In reality both intra- and inter-pocket scatterings are present, and the situation is best illustrated by a model calculation. The theoretical results are presented in Fig. 6c,d for an attractive impurity (that is, with negative scattering potential V imp =−1.5 eV). One can see a close similarity to the experimental data. We emphasize that such a feature is a unique property of s ± pairing gap. It is absent, for example, if we assumed an s ++ pairing instead. We also notice that the asymmetry in the impurity-DOS is linked to the band structure as well as the sign of the impurity potential. The negative sign for the impurity potential is consistent with the fact that there are more d-electrons on the Cu impurity site experimentally. Finally we should mention that the energy of the in-gap states could reach zero but only at a very specific value of the impurity potential neither in the Born nor the unitary limit. Therefore, the generic feature is the appearance of finite-energy in-gap states, as seen in our experiment. Our theoretical calculations based on the scalar scattering potential can really capture the main features of the experimental data, this gives further support and validates the observation of in-gap states by the non-magnetic Cu impurities. Taking into account the fact that the gaps are almost isotropic (Δ≈5 meV) on both the hole and the electron Fermi pockets [36] , [37] , we can exclude the nodal gap in the present system. Therefore, the observation of the in-gap states on non-magnetic Cu impurities here indicates a sign reversal of the superconducting gap, which gives an only choice of the s ± pairing. Sample synthesis and characterizations High quality Na(Fe 0.97 Co 0.03 )As and Na(Fe 0.97− x Co 0.03 T x )As (T=Cu and Mn) single crystals were synthesized by the self-flux method. Firstly, NaAs was prepared as the precursor. The Na (purity 99%) was cut into pieces and mixed with As powders (purity 99.99%), the mixture was put in an alumina crucible and sealed in a quartz tube in vacuum. The mixture was slowly heated to 200 °C and held for 10 h, followed by cooling down to room temperature. Then the resultant NaAs, and Fe (purity 99.9%), Co (purity 99.9%), T (Cu or Mn) (purity 99.9%) powders were weighed with an atomic ratio of NaAs:Fe:Co:T=4:(0.97− x ):0.03: x and ground thoroughly. The mixture was pressed into a pellet and loaded into an alumina crucible, sealed in an iron tube under Ar atmosphere. Then it was placed in the furnace and heated up to 950 °C and held for 10 h, followed by cooling down to 600 °C at a rate of 3 °C per h to grow single crystals. In the preparation process, the weighing, mixing and grounding were conducted in a glove box under argon atmosphere with the O 2 and H 2 O below 0.1 p.p.m. The DC magnetization measurement was carried out with a SQUID-VSM-7T (Quantum Design) with a resolution of 5 × 10 −8 emu. The resistivity measurement was done on a PPMS-16T (Quantum Design) with the standard four-probe method. STM/STS measurements The scanning tunnelling spectra were measured with an ultrahigh vacuum, low temperature and high magnetic field scanning probe microscope USM-1300 (Unisoku Co., Ltd.). The samples were cleaved at room temperature in an ultrahigh vacuum with a base pressure better than 1.5 × 10 −10 torr. In all STM/STS measurements, Pt/Ir tips were used. To lower down the noise of the differential conductance spectra, a typical lock-in technique with an ac modulation at 987.5 Hz was used. How to cite this article: Yang, H. et al. In-gap quasiparticle excitations induced by non-magnetic Cu impurities in Na(Fe 0.96 Co 0.03 Cu 0.01 )As revealed by scanning tunnelling spectroscopy. Nat. Commun. 4:2749 doi: 10.1038/ncomms3749 (2013).